Ultra-selective uranium separation by in-situ formation ofπ-fconjugated 2D uranium-organic framework With the rapid development of nuclear energy, problems with uranium supply chain and nuclear waste accumulation have motivated researchers to improve uranium separation methods. Here we show a paradigm for such goal based on the in-situ formation of π - f conjugated two-dimensional uranium-organic framework. After screening five π -conjugated organic ligands, we find that 1,3,5-triformylphloroglucinol would be the best one to construct uranium-organic framework, thus resulting in 100% uranium removal from both high and low concentration with the residual concentration far below the WHO drinking water standard (15 ppb), and 97% uranium capture from natural seawater (3.3 ppb) with a record uptake efficiency of 0.64 mg·g −1 ·d −1 . We also find that 1,3,5-triformylphloroglucinol can overcome the ion-interference issue such as the presence of massive interference ions or a 21-ions mixed solution. Our finds confirm the superiority of our separation approach over established ones, and will provide a fundamental molecule design for separation upon metal-organic framework chemistry. In response to the long-term energy crisis, the development of new energies is now becoming a hot topic. Nuclear energy, because of its high energy density and low carbon pollution, is thus viewed to be one of the effective alternatives [1] , [2] , [3] , [4] , [5] . However, the sustainable development of nuclear energy is still severely limited by the shortage and insufficient supply chain of uranium. On the other hand, the extensive use of radioactive uranium will also bring serious safety issue, such as environmental pollution and unexpectable diseases [6] . Thereby, it is important to carry out the research of uranium separation from used or new sources [7] , [8] , [9] , [10] , [11] , [12] , [13] . Spent fuel, as a typical used source, remains 93.4% unreacted uranium, which thereby can be as a major uranium source through separation, however, such separation was often blocked by the competing adsorption from a broad of metal ions, especially these physically and chemically similar f -block ions such as rare earth and other actinide ions [14] , [15] , [16] . Alternatively, seawater reserves abundant uranium, however, the ultralow uranium content down to 3 ~ 4 ppb and the serious vanadium ion interference still prevents the acquisition of uranium from seawater [17] , [18] , [19] , [20] , [21] , [22] , [23] , [24] , [25] . Therefore, significant effort should be devoted to improve uranium separation methods to meet the actual demand. As an analogue of graphene, 2D (two-dimensional) conjugated metal-organic frameworks (MOFs), are recently receiving increasing attentions, due to its uniqueness in both structure and properties, showing important applications in supercapacitors, batteries, thermoelectric devices, chemiresistive sensors and electrocatalysts [26] , [27] , [28] . The design and synthesis rule of such 2D materials has been realized by the in-plane integration between π -conjugated hexa-substituted aromatic cores and late transition metal ions in a square planar coordination geometry [29] , [30] , [31] . Inspired by such way, we can expect the construction of similar 2D π - f conjugated MOF through a comparable in-plane integration between UO 2 2+ ion with a planar coordination in f orbitals [32] , [33] , [34] and proper π -conjugated ligands, and further make a hypothesis in uranium separation upon such MOF assembly technology. In this regard, we show herein the molecule design and uranium separation route by means of the concept of in-situ formation of π - f conjugated uranium-organic framework (UOF). 2D MOF and ligand design Previous research has revealed the molecular design rule for conjugated 2D MOF [29] , [30] , [31] . The key was the in-plane coupling between metal ions and organic ligands in a defined and periodic manner. It was found that these metal ions such as Ni 2+ , Co 2+ , and Cu 2+ in the square planar coordination geometry and these hexa-substituted planar conjugated benzenes such as 1,3,5-triformylphloroglucinol (H 3 TFP) and 2,3,6,7,10,11-hexahydroxytriphenylene (H 6 HTP) meet the in-plane [3 + 2] coupling, where the organic ligands take the chelate coordination mode (model I and II, Fig. 1a ) and act as three-connecting nodes, while metal ions act as two-connecting linker, finally resulting in the π - d conjugated 2D MOF (Fig. 1b ) [35] , [36] . Different from these transition metal ions of Ni 2+ , Co 2+ , and Cu 2+ that use d orbit for coordination, UO 2 2+ ion, the common uranium type, affords the planar coordination feature in the f orbit and theoretically conducts more orbit to participate in coordination, generally showing the six-coordination fashion. Corresponding to this is the distinct coordination mode (model I and model II, Fig. 1c ) between organic ligands and UO 2 2+ ions and 2D MOFs generated by [3 + 2] or [3 + 3] coupling (Fig. 1d ), where UO 2 2+ ions act as three-connecting node and organic ligands act as two-connecting linker or three-connecting nodes, respectively. In this regard, we screened five comparable, planar conjugated ligands, composed of hexa-substituted H 3 TFP, H 6 HTP, and H 3 THQ (tetrahydroxyquinone), tetra-substituted H 2 HPD (2,5-dihydroxyterephthalaldehyde) and H 4 EAA (ellagic acid). As shown in Fig. 2 , all these substrates were found to be effective in UO 2 2+ capture from a 100 ppm UO 2 2+ solution after contacting for 24 h, giving a hierarchy of H 3 TFP (100%) > H 2 HPD (25.6%) > H 4 EAA (24.8%) > H 6 HTP (8.3%) > H 3 THQ (6%), implying H 3 TFP being the best one. Accordingly, the next investigation is just focused on H 3 TFP ligand. Fig. 1: Molecular design of conjugated 2D MOFs. a π - d in-plane integration in the manner of model I and II. b View of the π - d conjugated 2D MOFs by means of [3 + 2] coupling with π -conjugated organic ligand as three-connected node and metal ions in the square planar coordination geometry as two-connected linker. c π - f in-plane integration in the manner of model I and II. d View of the π - f conjugated 2D MOFs by means of [3 + 2] or [3 + 3] coupling with UO 2 2+ ion as three-connected node and π -conjugated organic ligand as two-connected linker or three-connected node. Full size image Fig. 2: Ligands used in this work. A screen of various organic ligands for UO 2 2+ capture upon in-situ formation of MOF method. The error bars indicate the standard deviation ( n = 3). Full size image To clarify the difference in UO 2 2+ capture for these organic ligands, we then carried out the calculation on the binding energy (ΔG) of these organic ligands with UO 2 2+ ion by density functional theory (DFT) method. A planar six-coordination model of one UO 2 2+ ion coordinated by three these organic ligands was used to carried out DFT calculation. The optimized coordination structures of them were shown in Supplementary Fig. 1 . The binding energy ( ΔG ) gives a hierarchy of H 4 THQ (−0.29 eV)>H 6 HTP (−0.69 eV)>H 4 EAA (−1.02 eV)>H 2 HPD (−2.99 eV)>H 3 TFP (−3.91 eV). Generally, negative binding energy ( ΔG ) suggests the reaction thermodynamically spontaneous, while this also obeys a rule, viz . the more negative, and the stronger the binding. Thus, the negative ΔG values mean that all these organic ligands can capture UO 2 2+ ion through coordination, which is consistent with the experimental results, while the smallest and biggest ΔG value in, respectively, H 3 TFP and H 4 THQ means the strongest and weakest binding and consequently the biggest and smallest UO 2 2+ uptake, which is also in good agreement with the experimental results. Moreover, the hierarchy in binding energy ( ΔG ) is also in accord with the hierarchy in the UO 2 2+ uptake, confirming the adsorption of UO 2 2+ ions by these organic ligand obeying the defined planar coordination principle. In addition, seen from the optimized coordination structures of them, it is found that the chelate coordination from the combination of one aldehyde oxygen and one hydroxyl oxygen (such as H 4 TFP and H 2 HPD) is more beneficial for strengthening U-O coordination and planar coordination configuration over the chelate coordination from two hydroxyl oxygens (such as H 4 EAA, H 6 HTP, H 4 THQ), due to steric hindrance effect. And this could be the key to determine the UO 2 2+ uptake performance. Moreover, the bigger conjugated organic molecule is beneficial for strengthening planar coordination configuration and consequently enhancing UO 2 2+ uptake, e.g., H 6 HTP and H 4 EAA vs. H 4 THQ. Adsorption kinetics Fast adsorption process is usually the way we want. We then tested the adsorption kinetics of H 3 TFP ligand from a 50 ppm U(VI) solution with pH = 3 through using 10 mg adsorbent (Fig. 3a ). Notably, the adsorption equilibrium was finished within 15 min with 100% removal efficiency, suggesting ultrafast adsorption kinetics, due to the thermodynamicly spontaneous chemical reaction through coordination assembly between UO 2 2+ ions and H 3 TFP ligand. After extending the contact time to 24 h and 48 h, we found that the residual uranium concentration was decreased down to ultralow level of 0.18 ppb and 0.15 ppb, respectively, far lower than the World Health Organization (WHO) standard (15 ppb) for uranium content in drinking water. In light of this data, the distribution coefficient, K d , was calculated up to 9.6 × 10 7 mL/g (a K d value exceeding 1.0 × 10 5 mL/g is usually considered as excellent adsorbent), implying strong affinity between adsorbents and uranium resulted from the strong U-O coordination interactions. This value ranks the top level among all established uranium adsorbents, including POP 1 -AO (1.1 × 10 6 mL/g) [37] , MIGPAF-13 (2.0 × 10 6 mL/g) [38] , SMON-PAO (3.7 × 10 5 mL/g) [39] , and PIDO/NF (2.8 × 10 5 mL/g) [7] . This exceptional uranium removal ability was further attested for a low concentration of U(VI) solution (1 ppm), giving a residual uranium concentration of 2.3 ppb after 5 min and 0.13 ppb after 48 h (Fig. 3b ), also far exceeding the WHO standard. Big K d value up to 2.1 × 10 6 mL/g was also observed. Fig. 3: Uranium adsorption upon H 3 TFP. a Adsorption kinetics from 50 ppm U solution upon H 3 TFP adsorbent. b Adsorption kinetics from 1 ppm U solution upon H 3 TFP adsorbent. c Adsorption capacity of H 3 TFP adsorbent. Highlight in blue represents the theoretical adsorption capacity. d A comparison in U uptake capacity between reported U adsorbents and our case. e Influence of interfering ions on U adsorption. f Selective U capture from a 21-ions mixture solution. The error bars indicate the standard deviation ( n = 3). Full size image Adsorption capacity Large adsorption capacity is also one of the goals pursued by adsorbent. Next, we investigated the adsorption capacity upon H 3 TFP adsorbent from a uranium solution with concentration of 10–1000 ppm. Interstingly, this adsorbent enabled 100% removal for all these uranium solutions (Fig. 3c ), which is never observed in the literature. The experimental uranium uptake capacity was as high as 1.0 g/g. If taking the formation of UOF through [3 + 3] coupling into account, the theoretical adsorption capacity is estimated as big as 1.6 g/g, which surpasses all established uranium adsorbents (Fig. 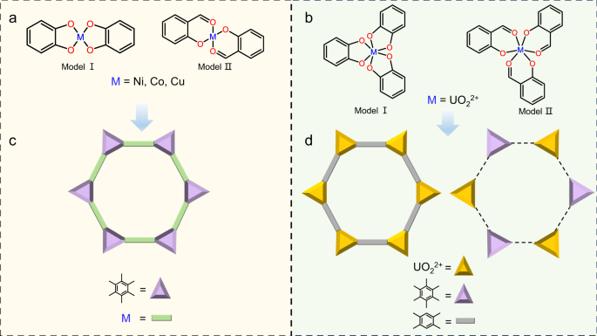Fig. 1: Molecular design of conjugated 2D MOFs. aπ-din-plane integration in the manner of model I and II.bView of theπ-dconjugated 2D MOFs by means of [3 + 2] coupling withπ-conjugated organic ligand as three-connected node and metal ions in the square planar coordination geometry as two-connected linker.cπ-fin-plane integration in the manner of model I and II.dView of theπ-fconjugated 2D MOFs by means of [3 + 2] or [3 + 3] coupling with UO22+ion as three-connected node andπ-conjugated organic ligand as two-connected linker or three-connected node. 3d , Supplementary Table 1 ) [40] , including these benchmark adsorbents such as MIL-101-DAMN (0.60 g/g) [41] , Cu-BTC (0.61 g/g) [42] , TFPPy-BDOH (0.98 g/g) [43] , and POP 3 -AO (1.07 g/g) [37] . This also confirmed the advantage of our method over established approaches. pH effect It was found that pH value showed significant effect on the uranium uptake performance (Supplementary Fig. 2 ). The optimal performance was found under pH = 3 and 5, whereas both increasing acidity and alkalinity would lead to sharp decrease in the uranium uptake, for example, 100% uranium removal under pH = 3 and 5 vs . 12.6% uranium removal under pH = 1 or 21.8% uranium removal under pH = 9. High acidity leading to a sharp decrease in uranium uptake is mainly due to the protonation that will significantly affect the coordination of H 3 TFP hydroxyl groups, and high alkalinity resulting in a sharp decrease in uranium uptake is mainly due to the solution of H 3 TFP under such condition that will significantly affect the UOF formation. Selectivity towards UO 2 2+ As we know, divalent copper and trivalent iron ion were found to construct 2D MOF with H 3 TFP ligands [35] , while the presence of trivalent 4f ions, or tetravalent thorium ion [23] , or vanadium ion were often found to give significant effect on UO 2 2+ capture [37] , [38] . Thereafter, it is important to research the uranium adsorption performance in the presence of these interfering ions. Then, we carried out the uranium adsorption experiments form a 10 ppm uranium solution under the presence of massive other interfering ions with U/M (M = Cu 2+ , Fe 3+ , Nd 3+ , Th 4+ , and VO 3 − ) ratio from 1:10 to 1:100 (Fig. 1e ). Notably, no decrease in the uranium uptake was observed in the presence of other interfering ions, even expanding the U/M ratio to 1:100, completely excluding the influence of interfering ions. Such selectivity towards UO 2 2+ ion over other ions is highly rare in the literature [44] , [45] . Furthermore, we carried out a selectivity test from a 21-ions mixture solution, including in Na + , K + , Cs + , Mg 2+ , Ca 2+ , Sr 2+ , Zn 2+ , Cd 2+ , Pd 2+ , Mn 2+ , Cu 2+ , Co 2+ , Ni 2+ , Cr 3+ , Fe 3+ , La 3+ , Gd 3+ , Nd 3+ , Th 4+ , UO 2 2+ , and VO 3 - (Fig. 1f ). It was found that UO 2 2+ was 100% captured, whereas other ions just gave less than 10% removal efficiency, suggesting highly selective capture of UO 2 2+ ion over other 20 ions. The selectivity of UO 2 2+ over Fe 3+ , Nd 3+ , Th 4+ , and VO 3 − can be easy to understand, since UO 2 2+ is planarly coordinated and can effectively construct the π-f conjugated 2D uranium-organic framework, whereas other ions such as Fe 3+ , Nd 3+ , Th 4+ , and VO 3 − are spherical coordinated and can not construct corresponding π-d/f conjugated 2D metal-organic framework. However, Cu 2+ ions own the planar coordination feature, and can form the π-d conjugated 2D metal-organic framework, which will theoretically result in considerably competitive adsorption with UO 2 2+ ion. Thereby, to understand the UO 2 2+ /Cu 2+ selectivity in this work, DFT calculation on binding energy was carried out (Supplementary Fig. 3 ). The negative binding energy ( ΔG ) of −1.16 eV implies the adsorption potential of H 3 TFP ligand towards Cu 2+ ions. But the binding towards Cu 2+ ion is far weaker than that towards UO 2 2+ ion, as evidenced by the ΔG value (−1.16 eV) in Cu 2+ ion that is far bigger than that (−3.91 eV) in UO 2 2+ ion; thus H 3 TFP ligand can enable selective UO 2 2+ capture over Cu 2+ ion. Recycle use and liquid-liquid extraction More interestingly, H 3 TFP adsorbent can be conveniently recovered in the form of precipitate through using 3 M HNO 3 as eluent, while the adsorbed uranium on adsorbent can be 100% desorbed into solution in the form of UO 2 (NO 3 ) 2 , possibly due to a disassembly of UOF with the breakage of all U-O coordination bonds. Such complete solid-liquid separation (Fig. 4 ) facilitates our following recycle use to an ideal form, as evidenced by observation of no decrease in both uranium adsorption and adsorbent recovery from a 100 ppm uranium solution after repeating adsorption-desorption cycles (Fig. 4 ) for 11 times (Supplementary Fig. 4 ). Fig. 4: Our MOF routes. View of the adsorption-desorption cycle by means of our separation approach in both solid- and liquid-extraction routes. Full size image Interestingly, although H 3 TFP is insoluble in water, however it gave good solubility in many organic solvents, involved in dichloromethane (DCM), toluene (PhMe), ortho-dichlorobenzene (ODCB), p-xylene (PX), m-xylene (MX), ortho-xylene (OX), and trimethylbenzene (TB). Thus, we further developed the liquid-extraction route (Fig. 4 ) and the results were shown in Supplementary Fig. 5 . Notably, such liquid-extraction route was found to be also effective for uranium capture. Especially, H 3 TFP in DCM and ODCB was found to give 100% removal for a 50 ppm uranium solution within 15 min. This result is comparable with that observed in the solid-extraction route. We also extended the contacting time up to 48 h for H 3 TFP in DCM, and found low residual concentration of uranium (1.24 ppb), which is also far below the WHO standard of drinking water. In both solid- and liquid-extraction routes, a key step in the desorption process is the solid-liquid separation between UO 2 (NO 3 ) 2 solution and H 3 TFP precipitation regeneration from desorption. Thus, it is important to reveal the solubility of H 3 TFP in water. As shown in Supplementary Fig. 6 , it was clear that H 3 TFP is completely soluble in ODCM, but insoluble in water. This can be further attested by UV-visiblespectral test (Supplementary Fig. 7 ), where H 3 TFP in ODCM gave a strong adsorption peak at 320 nm, while no obvious adsorption was observed for H 3 TFP in water. Extraction of uranium from seawater To confirm the practical application of our uranium separation method, we further explored uranium capture performance from natural seawater. It was found that the use of 10 mg H 3 TFP adsorbent can reduce a 10 L natural seawater (3.3 ppb U) to 0.1 ppb after contacting for 5 days, showing uranium uptake as high as 3.2 mg/g. If considering the time cost, the uranium uptake efficiency is 0.64 mg·g −1 ·d −1 . 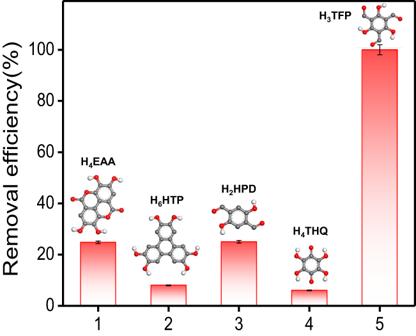Fig. 2: Ligands used in this work. A screen of various organic ligands for UO22+capture upon in-situ formation of MOF method. The error bars indicate the standard deviation (n= 3). Such value far exceeds the top adsorbents (Supplementary Table 2 ) such as PPH-OP (0.36 mg·g −1 ·d −1 ) [46] , AP-PIM-1 (0.32 mg·g −1 ·d −1 ) [47] , [48] , MIGPAF-13 (0.28 mg·g −1 ·d −1 ) [38] , and POP 1 -AO (0.15 mg·g −1 ·d −1 ) [37] . In addition, we also conducted the uranium extraction under a longer contacting time from a 20 L natural seawater (3.3 ppb U) using 10 mg H 3 TFP adsorbent. Impressively, 97% uranium can be captured after 10 days, giving uranium uptake as high as 6.4 mg/g, while extending contacting time up to 14 days did not increase uranium uptake. 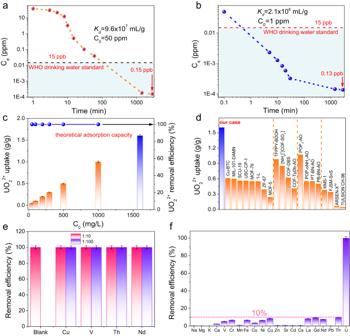Fig. 3: Uranium adsorption upon H3TFP. aAdsorption kinetics from 50 ppm U solution upon H3TFP adsorbent.bAdsorption kinetics from 1 ppm U solution upon H3TFP adsorbent.cAdsorption capacity of H3TFP adsorbent. Highlight in blue represents the theoretical adsorption capacity.dA comparison in U uptake capacity between reported U adsorbents and our case.eInfluence of interfering ions on U adsorption.fSelective U capture from a 21-ions mixture solution. The error bars indicate the standard deviation (n= 3). A comparison in uranium uptake between established materials and our case is shown in Supplementary Table 3 , which clearly suggests our case with the location of top level in the field of uranium extraction from seawater. Moreover, we should also consider the economy of uranium extraction from seawater. In generally, the manufacturing cost of adsorbents dominates the total cost for uranium extraction from seawater. For our case, the cost of preparing H 3 TFP adsorbent is as low as 1.3 $/g, confirming its economic feasibility. Such value is far below the current benchmark adsorbents such as COF 4 P (4.7 $/g) [14] and COF-4 (2.7 $/g) [15] . Uranium capture mechanism As mentioned above, the uranium capture upon H 3 TFP adsorbent majorly obeys the rule of in-situ formation of π - f conjugated 2D UOF, where the key is the assembly between π -conjugated H 3 TFP ligands and f ions of UO 2 2+ in the defined and periodic manner. The use of f orbit to participate in bonding for UO 2 2+ ions suggests the formation of considerably more ionic compounds than transition metals, meaning that UO 2 2+ ions are more likely to form crystalline MOFs than transition metals; [26] , [47] this can reasonably explain the selectivity of uranium over transition metal ions such as Cu 2+ and Fe 3+ , even though these metal ions can also form π - d conjugated 2D MOFs. The f orbit in UO 2 2+ ion shows the in-plane coordination feature, meeting the in-plane assembly, whereas other f ions such as rare-earth (trivalent state) and thorium (tetravalent state) ions afford sphere coordination feature [49] , [50] , which fully excludes the in-plane assembly; this can reasonably explain the selectivity of uranium over Nd 3+ and Th 4+ ions. Similarly, vanadium ions also own the sphere coordination feature, thus excluding the in-plane assembly and finally leading to the big selectivity of UO 2 2+ over VO 3 − ion. To confirm the formation of π - f conjugated 2D UOF during the uranium adsorption upon H 3 FTP adsorbent, we carried out a series of characterizations on the uranium-loaded samples (namely UOF-TFP), including in IR (infrared spectrum), XPS (X-ray photoelectron spectroscopy), PXRD (powder X-ray diffraction), TG (thermogravimetric analysis), N 2 adsorption, SEM-EDS (scanning electron microscope plus energy-dispersive X-ray spectroscopy), and TEM (transmission electron microscope). IR spectra disclosed new peak at 922 cm −1 , belonging to the antisymmetric vibration of uranyl ions, which, relative to UO 2 (NO 3 ) 2 ·6H 2 O with peak at 960 cm −1 (Supplementary Fig. 8 ) [44] , [45] , shows big red shift, implying strong coordination interactions between H 3 TFP adsorbent and uranyl ions. And coordination with the participation of both aldehyde and phenolic groups of H 3 TFP adsorbent can be further read out from IR peaks showing big shift or almost disappearance for aldehyde and phenolic groups, relative to free H 3 TFP molecule. The success in uranium capture upon H 3 TFP adsorbent can be further reflected in XPS spectrum, showing typical UO 2 2+ peaks at 381.8 eV and 392.7 eV for U4f 7/2 and U4f 5/2 , respectively (Supplementary Fig. 9 ). The values are significantly lower than that of UO 2 (NO 3 ) 2 ·6H 2 O (382.5 eV and 393.4 eV) [46] , [47] , also confirming the strong coordination interactions between H 3 TFP ligands and UO 2 2+ ions. The presence of two satellite peaks at higher binding energy, relative to U4f 7/2 and U4f 5/2 , confirms the U(VI) oxidation state in UOF-TFP. The single crystal of UOF-TFP can not be obtained, blocking us to access its exact structure. But, we can simulate its structure from powder X-ray diffraction (PXRD) plus pawley refinements [44] , [45] . PXRD pattern showed high crystallinity of UOF-TFP. In light of the coordination feature of both UO 2 2+ ions and H 3 TFP ligands, we then proposed a 2D MOF model, and then Pawley refinements were carried out on the experimental PXRD (Fig. 5a ). It was found that the refined PXRD pattern was in good agreement with the experimental counterpart, as evidenced by the small difference and reasonable R p = 2.65% and R wp = 3.78% values. The layered nets in UOF-TFP showed a staggered orientation (AB stacking). The structure of UOF-TFP was shown in Fig. 5b . UO 2 2+ ions afforded the planar six-coordination by three TFP 3− ligands using three phenolic oxygen and three aldehyde oxygen atoms. The TFP 3- ligands afforded a chelate coordination mode through using adjacent one phenolic oxygen and one aldehyde oxygen atom to fix one UO 2 2+ ion. The U-O bond length of 2.40–2.70 Å is in the normal range [33] , [34] . The π - f conjugated 2D net was built in a [3 + 3] way that each TFP 3− ligand connects to three UO 2 2+ ions, while each UO 2 2+ ion also connects to three TFP 3− ligands, resulting in an overall binodal hcb net. Moreover, such AB stacking led to small void among layers (Supplementary Fig. 10 ), occupied by water molecules. TG test disclosed the loss of solvent water molecules before 230 °C, and decomposition of UOF-TFP occurred after 310 °C (Supplementary Fig. 11 ). In addition, the micoporosity was confirmed by N 2 adsorption at 77 K (Supplementary Fig. 12 ). Fig. 5: Characterizations of UOF-TFP. a Experimental PXRD patterns and pawley refinements. b View of π - f conjugated 2D UOF-TFP. c SEM images and element mapping of UOF-TFP. d STEM-HADDF images and U element mapping of UOF-TFP. The highlight is the 2D hexagonal lattice of uranium ions. Full size image More impressively, such π - f conjugated 2D net can be intuitively read out by STEM-HADDF test. First, SEM disclosed the nanorod morphology of UOF-TFP (Fig. 5c ). EDS element analysis clearly disclosed the presence of uranium element, and the U/C atom ratio is well consistent with the structural data, confirming the accuracy of our structural simulation. Furthermore, such nanorod morphology can be also clearly read out from TEM images. Impressively, UO 2 2+ ions and its location can be clearly read out from STEM-HADDF images (Fig. 5d ), where the UO 2 2+ ions are approximately arranged in a hcb fashion with a distance of ca. 0.9 nm between two adjacent U ions, which is similar to that observed in the simulated structure data with a distance of ca. 0.81 nm. In addition, to gain deep insight into the local coordination sphere of the uranium species, U K-edge X-ray absorption near-edge structure (XANES, Supplementary Fig. 13 ) and extended X-ray absorption fine structure (EXAFS, Supplementary Fig. 14 ) spectroscopy were performed. UO 2 (NO 3 ) 2 ·6H 2 O was used as the reference standard. It was found that UOF-TFP rendered comparable XANES and EXAFS spectra with that observed in UO 2 (NO 3 ) 2 ·6H 2 O, confirming their similarity in the valence state and coordination surrounding of uranium. As we know, uranium in UO 2 (NO 3 ) 2 ·6H 2 O is hexavalent in the form of UO 2 2+ , and UO 2 2+ in UO 2 (NO 3 ) 2 ·6H 2 O takes planar six coordination with two NO 3 - ions and two coordination water molecules, where each NO 3 − ion displays a chelate coordination mode with two NO 3 − oxygen atoms to fix one UO 2 2+ ion. 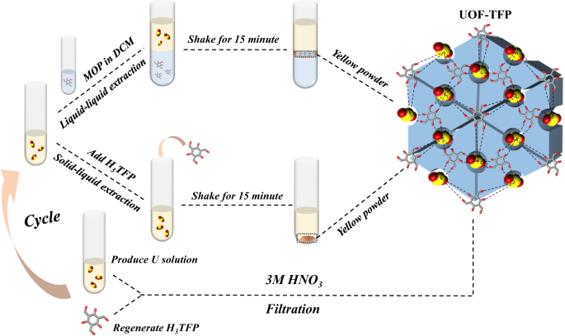Fig. 4: Our MOF routes. View of the adsorption-desorption cycle by means of our separation approach in both solid- and liquid-extraction routes. 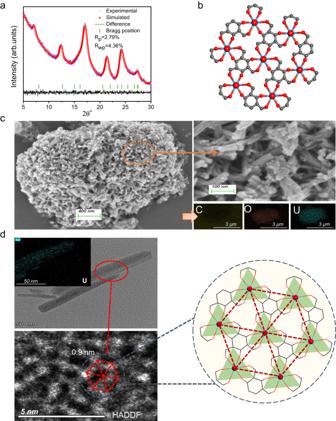Fig. 5: Characterizations of UOF-TFP. aExperimental PXRD patterns and pawley refinements.bView ofπ-fconjugated 2D UOF-TFP.cSEM images and element mapping of UOF-TFP.dSTEM-HADDF images and U element mapping of UOF-TFP. The highlight is the 2D hexagonal lattice of uranium ions. 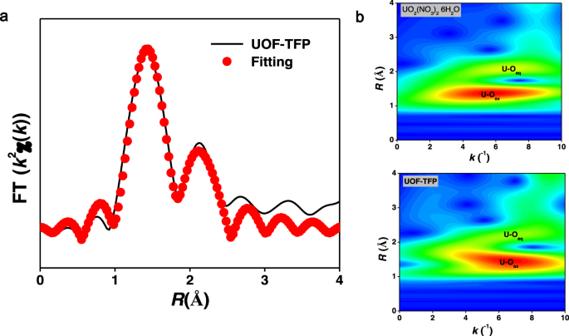Fig. 6: EXZAF of UOF-TFP. aExperimental EXZAF data (red) and fitting results (black).bView of coordination surrounding of UOF-TFP and UO2(NO3)2·6H2O, where U-Oaxrepresents the U = O coordination bonds, U-Oeqrepresents the U-OnitrateplusU-Owaterin UO2(NO3)2·6H2O and U-OhydroxylplusU-Oaldehydein UOF-TFP. Accordingly, we can deduce UO 2 2+ ions with the planar six coordination in UOF-TFP (Supplementary Table 4 ). High-quality fits of the EXAFS data for UOF-TFP (Fig. 6a, b ) strongly suggest an eight coordination of uranium, where two U-O coordinations with bond length of 1.85 ± 0.01 Å are assigned to U = O bond of UO 2 2+ ion, other six U-O coordinations with longer bond length are assigned to the planar U-O coordination from TFP 3- ligand. This also reveals two types of U-O bond with equal numbers in the bond length of 2.42 ± 0.02 Å and 2.51 ± 0.01 Å, respectively. We then comparied the results from EXAFS data with the results from structural simulation, and found that the U = O bond of UO 2 2+ ion form EXAFS data is well consistent with the results from structural simulation (1.84 Å), while the bond length of 2.42 ± 0.02 Å and 2.51 ± 0.01 Å from EXAFS data is close to U-O hydroxyl bond (2.40 Å, hydroxyl oxygen of TFP 3− as coordination atom) and U-O aldehyde bond (2.70 Å, aldehyde oxygen of TFP 3− as coordination atom) from structural simulation. Thereby, the structure of UOF-TFP can be once again confirmed by EXAFS results. Fig. 6: EXZAF of UOF-TFP. a Experimental EXZAF data (red) and fitting results (black). b View of coordination surrounding of UOF-TFP and UO 2 (NO 3 ) 2 ·6H 2 O, where U-O ax represents the U = O coordination bonds, U-O eq represents the U-O nitrate plus U-O water in UO 2 (NO 3 ) 2 ·6H 2 O and U-O hydroxyl plus U-O aldehyde in UOF-TFP. Full size image In summary, we have demonstrated a proof-of-concept of in-situ formation of π - f conjugated 2D UOF for targeting at highly efficient and selective uranium separation. Taking both coordination and self-assembly chemistry into account, through using the simple but powerful organic ligand of H 3 TFP molecule, we can easily appoint the self-assembly between π -conjugated H 3 TFP ligands and in-plane coordinated f UO 2 2+ ions in a defined and periodic manner, leading to the rapid and massive formation of UOF. Such feature finally offered an ideal uranium separation process, as evidenced by its superior performance, including in recorded theoretical uptake capacity, ultrafast adsorption kinetics, large distribution coefficient, big selectivity, and long-term repeatability. This work not only outlines a concept of how to use MOF chemistry to solve practical problems, but also points out a promising direction in the field of uranium separation. Materials and measurements H 3 TFP (99%), H 2 HPD (99%) and H 6 HTP (99%) were purchased from Jilin Chinese Academy of Sciences - Yanshen Technology Co., Ltd. H 4 THQ (99%), H 4 EAA (99%), UO 2 (NO 3 ) 2 ·6H 2 O (99%), and these organic solvents (99%) were purchased from Aladdin Biochemical Technology Co., Ltd. These were used as received without further purification. X-ray powder diffraction were collected by a Bruker AXSD8 Discover powder diffractometer at 40 kV, 40 mA for Cu Kλ (λ = 1.5406 Å). The simulated powder patterns were calculated by Mercury 1.4. Infrared Spectra (IR) were measured by a Bruker VERTEX70 spectrometer in the 700–3600 cm −1 region. The gas adsorption isotherms were collected on a Belsorp-max. Ultrahigh-purity-grade (>99.999%) N 2 gases were used during the adsorption measurement. The analyses of concentrations of U ions in the solution was carried out by ThermoFisher iCap7600 ICP-OES or iCap RQplus ICP-MS instruments. X-ray photoelectron spectra (XPS) were collected by Thermo Scientific ESCALAB 250 Xi spectrometer. Scanning electron microscopy (SEM) images were recorded on a Hitachi SU 8100 Scanning Electron Microscope. Transmission Electron Microscope (TEM) was recorded on a Talos F200x from Thermo Fisher Scientific. UV-vis spectroscopy were recorded at room temperature on a SHIMADZU UV-2700 spectrophotometer.